Long distance spin communication in chemical vapour deposited graphene Graphene is an ideal medium for long-distance spin communication in future spintronic technologies. So far, the prospect is limited by the smaller sizes of exfoliated graphene flakes and lower spin transport properties of large-area chemical vapour-deposited (CVD) graphene. Here we demonstrate a high spintronic performance in CVD graphene on SiO 2 /Si substrate at room temperature. We show pure spin transport and precession over long channel lengths extending up to 16 μm with a spin lifetime of 1.2 ns and a spin diffusion length ∼ 6 μm at room temperature. These spin parameters are up to six times higher than previous reports and highest at room temperature for any form of pristine graphene on industrial standard SiO 2 /Si substrates. Our detailed investigation reinforces the observed performance in CVD graphene over wafer scale and opens up new prospects for the development of lateral spin-based memory and logic applications. Two-dimensional atomic crystals represent a new class of nanoscale materials for fundamental studies and potential applications in future electronics. Since the discovery of graphene, its superlative transport properties and their prospects in the field of nanoelectronics have been demonstrated [1] . Graphene also remains at the forefront for spintronic applications, being ideal for long-distance spin communication [2] . Owing to the low intrinsic spin–orbit coupling and negligible hyperfine interaction, the proposed spin coherence length ( λ s ) in graphene can extend up to 100 μm with spin lifetime ( τ s ) ∼ 1 μs [3] , [4] , [5] . Spin-logic technologies [6] aim to harness this giant spintronic potential for manipulating nanomagnets [7] via spin currents transmitted over long graphene channels. This will potentially bring novel developments in spintronic device designs from the conventional giant magnetoresistance (GMR) and tunnel magnetoresistance (TMR) structures where a spin transport of only few nanometre distance is used [6] , [8] . The realization of these functionalities can lead to all-spin-logic and memory devices with high performance and low power consumption [6] . Pioneering experiments [9] and subsequent important studies [10] , [11] , [12] , [13] , [14] , [15] , [16] on pure spin transport showed λ s ∼ 2 μm with τ s in the range of 100–770 ps for exfoliated graphene on Si/SiO 2 substrate [9] , [10] , [11] , [12] , [13] , [14] , [15] , [16] , [17] , [18] , [19] . Although chemically modified graphene such as hydrogenated graphene has been reported to show enhanced λ s ∼ 7 μm and τ s ∼ 2.7 ns [20] , hydrogenation leading to colossal spin–orbit coupling [21] with reduced λ s ∼ 1 μm and τ s ∼ 90 ps, and additional spin relaxation by created magnetic moments [22] have also been reported. Even though extremely large values of λ s and τ s were estimated in epitaxial graphene on SiC substrates via magnetoresistance measurements [23] , the pure spin transport experiments revealed values for λ s and τ s up to 2 μm and 2 ns, respectively [24] , [25] . High-mobility exfoliated graphene on atomically flat hexagonal boron nitride (h-BN) substrates and suspended graphene structures [2] , [15] , [26] have been employed for enhanced spin parameters, with τ s ∼ 150–400 ps and λ s reaching up to 4.7 μm. More recently, spin diffusion length nearly double in magnitude with nanosecond spin lifetime in high-quality h-BN encapsulated exfoliated graphene structures [27] , [28] have also been acheived. Most of these studies were performed using exfoliated flakes of graphene and h-BN due to their higher quality, but their size limitation to few micrometres has severely restricted any practical applicability. Out of the different approaches to produce large-area graphene, chemical vapour deposition (CVD) is by far the most viable and industry compatible technique [29] , [30] , [31] , [32] . Such large area wafer scale graphene can be transferred to desired substrates, patterned and modified locally, achieving different electronic functionalities for the much anticipated all-graphene circuits [33] , [34] . Compared with exfoliated graphene, the electronic quality of the CVD form is seen to be compromised by polycrystalline domains, wrinkles, ripples, foreign contaminations, inter-grain connectivity and strain fields due to graphene–substrate interaction, introduced during the growth and subsequent transfer process [31] , [35] , [36] , [37] , [38] , [39] . Some of these features affect the charge transport substantially and thus can potentially alter the spin transport in CVD graphene. The challenges involved in CVD graphene device processing and their effect on sensitive spin currents so far resulted in fewer reports with spin parameters limited to τ s ∼ 200 ps and λ s ∼ 2 μm with channel length up to 4 μm on Si/SiO 2 substrates at room temperature [12] , [40] , [41] , [42] . Even though theoretical studies advocate larger spin lifetimes on SiO 2 substrates [39] with spin transport being less influenced by imperfections such as grain boundaries or ripples in CVD graphene [43] and flexural distortions [44] , studies involving microscopic descriptions [37] , [45] attribute a greater role of grain boundaries in relaxation. The later studies [37] , [45] indicate that achieving improved grain connectivity while decreasing impurities during the transfer and fabrication processes is key to enhanced charge and spin transport in CVD graphene. These facts point out that there exists an immense potential for long-distance spin transport in large-scale CVD graphene on SiO 2 /Si substrate, which remains a challenge to be realized experimentally. In this study, we demonstrate the long-distance spin transport capability of CVD graphene in channels extending up to 16 μm on SiO 2 /Si substrate at room temperature. Pure spin transport and precession measurements in such long channels give rise to a spin lifetime of 1.2 ns with spin diffusion length ∼ 6 μm, which are the highest values obtained so far for any form of pristine graphene on SiO 2 /Si substrates at 300 K. Comprehensive measurements with various channel lengths and gate voltages performed at different temperatures enable us to understand the spin-scattering mechanism and evolution of the spin parameters in CVD graphene. The demonstration of long-distance spin transport in CVD graphene constitutes a major advancement for lateral spintronic memory and logic technologies. Device and measurement A schematic representation of a device along with the nonlocal (NL) technique for measurement of spin signal is shown in Fig. 1a . Spin polarization in CVD graphene is created by electrical spin injection (current I ) from a ferromagnetic tunnel contact and the pure spin transport signal (voltage V ) is detected by a similar contact placed nonlocally at a distance L. A modulation in the NL spin signal with magnetic field gives an estimate of induced spin polarization, and other spin parameters such as the spin lifetime τ s and diffusion length λ s in graphene. Essentially, two kinds of measurements are performed in all our CVD graphene devices having different channel lengths. First, the spin injection efficiency and spin transport distance are evaluated from spin valve measurement, where an in-plane magnetic field ( B ‖ ) parallel to the ferromagnetic electrodes is swept to measure the change in pure spin signal between parallel and antiparallel configurations of magnetizations of the ferromagnetic electrodes. Next, the spin lifetime τ s , diffusion constant D s and diffusion length λ s are obtained by Hanle measurement, in which an out-of-plane magnetic field ( B ⊥ ) perpendicular to the magnetization of ferromagnetic electrodes is swept to obtain continuous variation in spin signal due to spin precession. Devices having long CVD graphene channels with ferromagnetic tunnel contacts (TiO 2 /Co) were fabricated to achieve long-distance spin transport. We employed large-area CVD graphene grown on copper foil, which was transferred onto SiO 2 /Si substrate and patterned into long channels. The ferromagnetic tunnel contacts were prepared by electron beam lithography and liftoff techniques. The TiO 2 barrier in the tunnel contacts was prepared by an evaporation of 8 Å of Ti and oxidation in an oxygen atmosphere. Subsequently, 65 nm of Co and a capping layer of 4 nm of Al were deposited by electron beam evaporation. The details of the device fabrication process are described in the Methods section. An optical microscope image of a fabricated device with 16-μm-long graphene channel and multiple TiO 2 /Co contacts is presented in Fig. 1b . 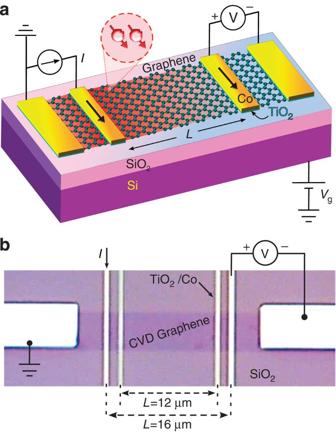Figure 1: CVD graphene field effect device for pure spin transport. (a) Schematic representation of a graphene device with ferromagnetic tunnel contacts for spin injection and detection in NL geometry. The current (I) injection circuit creates spin polarization in graphene via electrical spin injection and the isolated voltage (V) measurement circuit probes the NL pure spin signal. The red colour represents the spin density, which diffuses away from the place of injection in the graphene channel. The highly doped Si with SiO2layer is used as the back gate to control the carrier density (n) in graphene. (b) Optical microscope image of a fabricated long channel CVD graphene device on SiO2/Si substrate with multiple ferromagnetic tunnel contacts of Co/TiO2patterned by electron-beam lithography. The NL measurement scheme is presented for 16-μm-long graphene channel with current (I) and voltage (V) circuits. The spin transport measurements were performed using DC currents, in the temperature range of 4.2–300 K. Figure 1: CVD graphene field effect device for pure spin transport. ( a ) Schematic representation of a graphene device with ferromagnetic tunnel contacts for spin injection and detection in NL geometry. The current ( I ) injection circuit creates spin polarization in graphene via electrical spin injection and the isolated voltage ( V ) measurement circuit probes the NL pure spin signal. The red colour represents the spin density, which diffuses away from the place of injection in the graphene channel. The highly doped Si with SiO 2 layer is used as the back gate to control the carrier density ( n ) in graphene. ( b ) Optical microscope image of a fabricated long channel CVD graphene device on SiO 2 /Si substrate with multiple ferromagnetic tunnel contacts of Co/TiO 2 patterned by electron-beam lithography. The NL measurement scheme is presented for 16-μm-long graphene channel with current ( I ) and voltage ( V ) circuits. Full size image Structural and electrical characterization of CVD graphene To understand the quality of graphene channel and the TiO 2 /Co tunnel contacts, we performed detailed structural and electrical characterization of the devices. 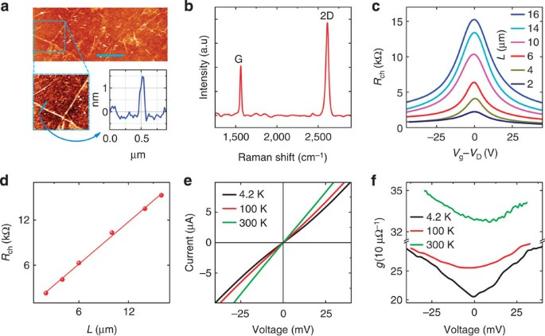Figure 2: Characterization of the CVD graphene and ferromagnetic tunnel contacts. (a) Atomic force microscope image of a graphene channel, with scale bar of 5 μm along with a magnified image of a ripple featuring region and its height profile scan. (b) Representative micro Raman spectrum of CVD graphene channel. (c) Graphene channel resistance (Rch) for different channel lengths as a function of gate voltage (Vg)–Dirac point (VD) (Dirac curves) at room temperature. (d) The linear enhancement of the resistance with graphene channel length atVg−VD=0. (e) Three-terminalI–Vcharacteristics of a Co/TiO2/graphene contact at different temperatures. (f) Differential conductanceg(dI/dV) plot of the contact as a function of bias voltage at different temperatures. Figure 2a displays an atomic force microscope image of the graphene channel in a device with relatively low density of ripples and resist residues on a region extending over 20 μm. Our optimized fabrication process ensured that the ripples introduced during the transfer process are sparse (height ∼ 1 nm shown in Fig. 2a ). Figure 2b shows a representative Raman spectrum of CVD graphene, where a dominant 2D peak is observed compared to the G peak confirming its single-layer nature. In addition, the D peak was found to be of negligible intensity, indicating a low sp 3 -type or vacancy defect density [46] . Raman spectra taken at different places in all graphene channels yielded similar results, indicating uniformity in the CVD graphene. Figure 2: Characterization of the CVD graphene and ferromagnetic tunnel contacts. ( a ) Atomic force microscope image of a graphene channel, with scale bar of 5 μm along with a magnified image of a ripple featuring region and its height profile scan. ( b ) Representative micro Raman spectrum of CVD graphene channel. ( c ) Graphene channel resistance ( R ch ) for different channel lengths as a function of gate voltage ( V g )–Dirac point ( V D ) (Dirac curves) at room temperature. ( d ) The linear enhancement of the resistance with graphene channel length at V g − V D =0. ( e ) Three-terminal I – V characteristics of a Co/TiO 2 /graphene contact at different temperatures. ( f ) Differential conductance g (d I /d V ) plot of the contact as a function of bias voltage at different temperatures. Full size image Next, the quality of the graphene was electrically assessed by the Dirac curves obtained from four probe channel resistance measured as a function of the gate voltage ( V g ). As shown in Fig. 2c , the resistance scales linearly with channel lengths, indicating a global uniformity of the CVD graphene. The carrier mobility evaluated from the Dirac curves was found to be ∼ 2,000 cm 2 V −1 s −1 with sheet resistance ∼ 5 kΩ/□ for different channels at room temperature. The similar sheet resistance of channels indicates a similar diffusion constant ( D c ) over a large area (see Supplementary Note 1 and Supplementary Table 1 ). The Dirac points ( V D ) were seen to lie in the range of −3 to −10 V, indicating a low doping of graphene. The typical temperature dependence of the Dirac curves of a graphene channel are shown in Supplementary Fig. 1 . It reveals a weak temperature dependence of graphene resistivity, indicating a dominating role of static scatterers. We obtain momentum scattering time τ p ∼ 20–50 fs and electron mean free path l mfp ∼ 20–50 nm (depending on the gate voltage) for all graphene channels. The low mean free path compared with the device dimension (several μm) along with a similar charge diffusion constant ( D c ) confirms the diffusive regime of electrical transport in CVD graphene (see Supplementary Note 1 and Supplementary Table 1 ). Grain boundaries in CVD graphene can contribute substantially to the residual resistance R ch (4.2 K) [37] , and the nature of impurities at the grain boundaries can further affect spin transport in CVD graphene. The grain size in the CVD graphene employed here was found to lie between 1 and 10 μm with median grain size ∼ 2 μm over a large scale. We also note that the grain concentration varied from device to device (as the device dimensions are comparable to the grain size, especially for shorter channels). In spite of this, we obtained a fairly linear dependence of resistance with length of the channel (shown in Fig. 2d ), indicating a low contribution of grain boundary scattering to the resistance. In addition, the low mean free path further indicates the dominance of intra-grain scattering to the momentum relaxation and thus the spin relaxation. Such intra-grain scattering can be attributed to substrate-induced disorder effects and defects induced during transfer process [39] , [45] . The interface resistance ( R i ) of the ferromagnetic tunnel contacts obtained from three-terminal measurements was found to be 4–5 kΩ at room temperature. Figure 2e shows typical nonlinear tunnelling current–voltage ( I–V ) characteristics of a TiO 2 /Co contact with weak temperature dependence. The corresponding differential conductance in Fig. 2f also shows a minimum at zero voltage at all the temperatures. These characteristics indicate the dominating tunnelling transport in Co/TiO 2 /graphene contacts [47] . The contact resistances R i are found to be of the order of the square resistance of graphene channel R Sq (see Supplementary Fig. 2 ) and can circumvent the conductivity mismatch problem [48] , [49] for spin injection. Long-distance spin transport and precession in CVD graphene To demonstrate the long-distance spin transport in CVD graphene, systematic measurements were performed on various channel lengths extending up to 16 μm. The spin valve and Hanle precession measurements were carried out in four-terminal NL configurations (as depicted in Fig. 3 ). Spin-polarized electrons are electrically injected from the ferromagnetic tunnel contact in the current circuit, which diffuse in the graphene channel and are detected by the NL voltage circuit. The isolated current and voltage circuits in the NL configuration ensure measurement of pure spin signals without spurious charge-related magneto-resistive contributions from ferromagnetic contacts or graphene channel. For an NL spin signal V = V NL measured at the detector (Det) with respect to reference electrode, an NL resistance is defined as R NL = V NL / I , with I being the current through the injector (Inj). A change in the magnetization configuration of the injector (Inj) and detector (Det) ferromagnets from parallel (↑↑ or ↓↓) to antiparallel (↑↓ or ↓↑) alignment leads to a spin valve signal change Δ V NL , characterized by an NL resistance change Δ R NL =Δ V NL / I . It is a measure of the spin splitting (Δ μ = μ ↑ − μ ↓ , with μ ↑ and μ ↓ being the chemical potentials of up (↑) and down (↓) spins, respectively) present in the graphene channel under the detector contact. The different shape anisotropies of the ferromagnets (Inj and Det) ensure different switching fields for the observation of spin valve signal by sweeping an in-plane magnetic field B ‖ . In Fig. 3a , we show the spin valve signal obtained on a graphene channel with L =16 μm at room temperature and a gate voltage V g =0 V. Spin valve signals with clear switching in such long channels have not been observed before in any form of pristine graphene on conventional Si/SiO 2 substrates at room temperature. The spin signals for channel lengths beyond 16 μm were dominated by noise in our measurements. 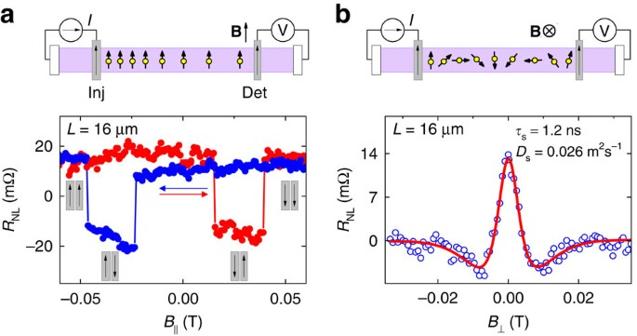Figure 3: Long-distance spin transport in CVD graphene device at room temperature. (a) NL spin valve signal with channel lengthL=16 μm with in-plane magnetic field (B‖) sweep as depicted in the figure. The high and low values of NL resistanceRNLcorrespond to the parallel (↑↑ or ↓↓) and antiparallel (↑↓ or ↓↑) configurations of the ferromagnetic injector (Inj) and detector (Det) electrodes, respectively. The blue and red colours indicate the direction of magnetic field sweep as represented by the arrows with respective colours. (b) NL Hanle spin precession signal obtained by a perpendicular magnetic field (B⊥) sweep in parallel configuration (↑↑) of ferromagnetic electrodes forL=16 μm graphene channel. The raw data points are fitted with the Hanle equation, to extract spin lifetimeτsand spin diffusion constantDs. Figure 3: Long-distance spin transport in CVD graphene device at room temperature. ( a ) NL spin valve signal with channel length L =16 μm with in-plane magnetic field ( B ‖ ) sweep as depicted in the figure. The high and low values of NL resistance R NL correspond to the parallel (↑↑ or ↓↓) and antiparallel (↑↓ or ↓↑) configurations of the ferromagnetic injector (Inj) and detector (Det) electrodes, respectively. The blue and red colours indicate the direction of magnetic field sweep as represented by the arrows with respective colours. ( b ) NL Hanle spin precession signal obtained by a perpendicular magnetic field ( B ⊥ ) sweep in parallel configuration (↑↑) of ferromagnetic electrodes for L =16 μm graphene channel. The raw data points are fitted with the Hanle equation, to extract spin lifetime τ s and spin diffusion constant D s . Full size image We further establish the spin transport in such long channels and evaluate the spin parameters through NL Hanle spin precession measurements ( Fig. 3b ). In the Hanle geometry, although the ferromagnetic electrodes are kept parallel, the injected spins undergo Larmor precession (frequency ; Landé g -factor g =2) about the perpendicular magnetic field ( B ⊥ ) resulting in a modulation of the detected spin signal. To evaluate the spin parameters (signal amplitude Δ R NL , lifetime τ s , diffusion length λ s , diffusion constant D s ), we fit the data with the empirical formula Eq. (1) encompassing the spin diffusion, precession and dephasing contributions [9] , [11] , [13] . where L is the effective channel length between the injector and the detector in our devices. The width W of the graphene channel is 5 μm and the measured graphene square conductivity σ s ∼ 200 μS. At 300 K, for V g =0 and L =16 μm, we obtain a spin lifetime of τ s =1.23±0.101 ns with spin diffusion constant D s =0.0264±0.002 m 2 s −1 , yielding a spin diffusion length λ s ∼ 6 μm. These values are the highest spin parameters achieved so far in CVD graphene and also in any form of pristine graphene on SiO 2 /Si substrate at room temperature. The parameters are also higher than the reports of high-quality exfoliated graphene on h-BN substrate [2] or suspended devices [15] , [26] and comparable to the most recent h-BN encapsulated high-quality exfoliated graphene devices [27] , [28] . Channel length dependence of the spin signal Systematic NL measurements were performed on various channel lengths L =2–16 μm at room temperature. 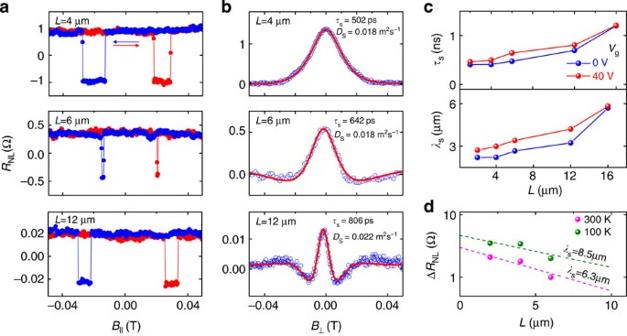Figure 4: Channel length-dependent spin transport in CVD graphene. (a) Spin valve measurements in device with different graphene channel lengths at room temperature andVg=0 V. (b) Hanle spin precession measurements at room temperature in device with different graphene channel lengths along with fitting with equation (1) and extracted spin parametersτsandDsatVg=40 V. (c) Spin lifetimeτsand spin diffusion lengthλswith graphene channelL=2–16 μm atVg=0 (blue circles) and 40 V (red circles) at room temperature as extracted from the Hanle fitting. (d) Length dependence of the spin signal and scaling fit () to spin signal for graphene channelL=2–6 μm on a device using one injection contact at 100 and 300 K forVg=0 V. Figure 4a shows representative spin valve and Hanle measurements for channel lengths of 4, 6 and 12 μm. The NL spin valve resistance Δ R NL is found to decrease for increasing channel lengths, from 4 Ω in L =2 μm to 20 mΩ in L =16 μm at room temperature. Figure 4b presents the corresponding Hanle data measured for different channels along with fits to equation (1). The extracted spin parameters from Hanle fits are found to be in the range of τ s =0.4–1.2 ns, D s =0.018–0.026 m 2 s −1 and λ s ∼ 3–6 μm for various channel lengths with V g =40 V at room temperature (see Supplementary Table 1 ). Note that for each channel the charge diffusion constants ( D c ) evaluated from the Dirac curves matched reasonably well with the spin diffusion constants ( D s ), which supports our current analysis. Although at a constant carrier density, small disparity and variations between the D c and D s are observed, including device to device variation, but the differences are very close and well within affordable limits ( D c =0.022±0.005) as widely reported [2] , [10] , [20] . We observe higher values of extracted τ s and λ s for longer graphene channels as presented in Fig. 4c . Notably, the longer channels increase the diffusion time, ensuring a higher accuracy in probing the graphene channel properties and hence the spin parameters. Such devices with longer channels also reduce the effect of contacts and dimensionality problems that can lead to possible underestimation of spin parameters [50] , [51] . Figure 4: Channel length-dependent spin transport in CVD graphene. ( a ) Spin valve measurements in device with different graphene channel lengths at room temperature and V g =0 V. ( b ) Hanle spin precession measurements at room temperature in device with different graphene channel lengths along with fitting with equation (1) and extracted spin parameters τ s and D s at V g =40 V. ( c ) Spin lifetime τ s and spin diffusion length λ s with graphene channel L =2–16 μm at V g =0 (blue circles) and 40 V (red circles) at room temperature as extracted from the Hanle fitting. ( d ) Length dependence of the spin signal and scaling fit () to spin signal for graphene channel L =2–6 μm on a device using one injection contact at 100 and 300 K for V g =0 V. Full size image To avoid any ambiguity, we also evaluated the spin parameters in an alternative way from the length dependence of the spin signal . Figure 4d shows the length dependence of the Δ R NL for L =2–6 μm graphene channels at 300 and 100 K for V g =0 V. It has to be noted that the measurements with L =2–6 μm belong to a single device with the same contact being used for spin injection. With a fairly good uniformity in the electronic quality of our CVD graphene over a large area, we obtained spin diffusion lengths λ s =8.5 and 6.3 μm at 100 and 300 K, respectively. We did not consider devices having different injector contacts or devices from different batches of fabrication, as they might lead to uncertainty arising out of varied contact properties. The spin diffusion length obtained here complements the results of the Hanle measurements ( λ s ∼ 6 μm) for the longest channel fairly well. Temperature and carrier density dependence of spin parameters We now present the detailed temperature and gate-dependent measurements showing the evolution of the spin transport in CVD graphene. The temperature dependence of spin parameters in devices with different channel lengths (shown in Fig. 5a,b ) indicates an increase in Δ R NL and τ s at lower temperatures. Such increase has also been observed in previous studies on exfoliated graphene crystals [11] . Similarly, enhancement of Δ R NL and τ s are also observed with increase in applied gate voltage V g (increased carrier concentration n in graphene) as displayed in Fig. 5c,d . Increased carrier concentrations can effectively reduce the spin–orbit coupling in graphene on SiO 2 substrate, as theoretically proposed recently [52] . This can significantly reduce the spin flip scattering and enhance the spin lifetime as observed in our devices. Such enhancement of Δ R NL and τ s can also be attributed to the competition between the resistances of graphene channel R ch and the tunnel contacts R i , as R ch is observed to decrease with gate voltage. A high R i is expected to prevent back diffusion of spins into the ferromagnet and faster spin relaxation [48] . The observed enhancement in Δ R NL and τ s in our case is in agreement with behaviour expected for relatively low resistive tunnel barriers ( R i ∼ R ch ) [10] , [53] . In addition, recent theoretical results based on spin–pseudo spin interaction in graphene also show reduction of spin parameter at low energy (closer to Dirac point) [54] . In convergence with theoretical predictions, the increasing trends of Δ R NL and τ s were reproducibly observed in all CVD graphene channels in our study. These observations also clearly indicate that the spin parameters at room temperature can be further enhanced with higher carrier density in graphene, which can be achieved by using ultra-thin gate dielectrics on graphene channels. The data presented here were measured using an injection current of 30 μA. No significant variation of either the Δ R NL or τ s was detected for bias currents in the range 5–50 μA. 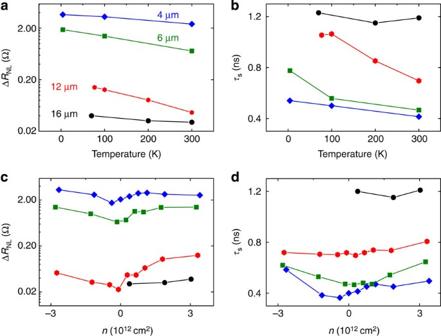Figure 5: Temperature and carrier density dependence of spin parameters. (a,b) Temperature (T) dependence of spin signal ΔRNLand spin lifetimeτsatVg=0 for different graphene channel lengths. (c,d) Carrier density (n) dependence of spin signal ΔRNLand spin lifetimeτsat room temperature. Carrier density (n) of graphene channel are controlled by application of back gate voltage (Vg) in the range of −40 V to +40 V. Colours represent the channel lengths:L=4 μm (blue), 6 μm (green), 12 μm (red) and 16 μm (black). Figure 5: Temperature and carrier density dependence of spin parameters. ( a , b ) Temperature ( T ) dependence of spin signal Δ R NL and spin lifetime τ s at V g =0 for different graphene channel lengths. ( c , d ) Carrier density ( n ) dependence of spin signal Δ R NL and spin lifetime τ s at room temperature. Carrier density ( n ) of graphene channel are controlled by application of back gate voltage ( V g ) in the range of −40 V to +40 V. Colours represent the channel lengths: L =4 μm (blue), 6 μm (green), 12 μm (red) and 16 μm (black). Full size image The observation of long distance spin transport ( L =16 μm) and enhanced spin parameters ( λ s =6 μm and τ s ∼ 1.2 ns) in CVD graphene on SiO 2 /Si substrate with reasonable mobility ( μ ∼ 2,000 cm 2 V −1 s −1 ) is quite striking and beyond expectations. It is also contrary to the conventional belief that such spin transport can only be realized in high-mobility single crystal graphene devices, structures with suspended schemes [15] , [26] , h-BN substrate [2] and encapsulation [27] , [28] schemes. However, the experimental outcomes [2] , [15] , [26] and recent theories do indicate that the SiO 2 substrate should not affect the spin parameters significantly [55] , [56] . It has also been demonstrated that a variation of mobility does not alter the observed spin lifetimes in graphene [57] . The ripples or wrinkles, which the CVD graphene features, are predicted and seen to weakly affect the spin parameters [43] , [44] . Corrugations and flexural distortions are also seen to set only the upper limit of spin lifetime in graphene [44] . Such extrinsic factors and in-plane defects predominantly show Elliot–Yafet (EY) relaxation [58] signature in graphene as reported previously [11] , [12] . However, the substrate disorder and surface ad-atoms [56] can locally enhance the Rashba spin–orbit coupling, leading to a substantial contribution of D’yakonov–Perel (DP) mechanism of spin relaxation [52] . A simple analysis of the dependence of spin relaxation time τ s on momentum relaxation time τ p (see Supplementary Note 2 and Supplementary Fig. 3 ) shows the contribution of both EY and DP mechanisms for spin relaxation in CVD graphene, which is similar to the latest study on exfoliated graphene [2] . However, we acknowledge that such phenomenological analysis on experimental data is far from theoretical perspectives and the microscopic origin of spin relaxation mechanisms in graphene still needs to be uncovered [5] . The primary source of spin relaxation remains an open question, as both EY and DP mechanism suggest theoretical τ s in the microsecond range [3] , [58] , [59] in contrast to the τ s ∼ 1 ns observed here and other graphene experiments. Instead, the recently proposed spin-flip exchange field from magnetic moments of impurity atoms or vacancies and magnetic impurities trapped at grain boundaries [60] , [61] can provide faster spin relaxation and can lead to practical τ s ∼ 1 ns, as observed in our experiments. More recently, for further understanding of spin relaxation in graphene in general, spin–orbit-induced entanglement of spin and pseudospin leading to spin relaxation in quasi-ballistic transport regime has also been proposed [54] . In addition to these proposed mechanisms, the role of ferromagnetic contacts and channel length as observed in our experiments should also be considered in theory for a more quantitative and precise understanding of spin relaxation in graphene [62] . In conclusion, we have demonstrated long-distance spin transport in CVD graphene channels with enhanced spin diffusion length and lifetime at room temperature. Employing 16-μm-long graphene channels, we observed a spin diffusion length ∼ 6 μm and spin lifetimes up to 1.2 ns at room temperature. The spin signal and lifetime showed further enhancements at higher gate voltages and lower temperatures. The spin parameters obtained in our experiments are up to six times higher than previous reports on CVD graphene and are also the highest reported values for any form of pristine graphene on SiO 2 substrate at room temperature. The comprehensive measurements and analysis showing enhanced spin parameters with graphene channel length give a further insight into the effect of contacts in spin relaxation. The accomplishment of long-distance superior spin transport in wafer-scale CVD graphene on SiO 2 substrate makes this study a vital step for future graphene spintronics technologies. With the recent reports of high-quality wafer-scale mono-domain CVD graphene [63] and the possibility to grow all CVD graphene/h-BN-encapsulated heterostructures, the spintronic functionalities in CVD graphene can take a giant leap in the near future. Our results will proliferate the development of long-distance spin communication in devices and circuits based on CVD graphene channels. Device Fabrication The CVD graphene spintronic devices are prepared on doped Si wafer with a thermally grown 285-nm-thick SiO 2 layer. The commercially procured CVD graphene (from Graphenea) was transferred onto the Si/SiO 2 substrate using a thicker polymethyl methacrylate (PMMA)-assisted wet transfer process [18] . The CVD graphene was then patterned by optical lithography into long stripes (20–30 μm) and the rest of the graphene was etched away by oxygen plasma with 50 W power for 30 s. This was followed by annealing in Ar/H 2 atmosphere at 400 °C, to remove possible resist residues. Ferromagnetic tunnel contacts (Co/TiO 2 ) were fabricated on the CVD graphene stripes with long channel lengths having multiple spacing ( L =2–20 μm) for studying the length dependence of the spin signal. The patterning for the ferromagnetic tunnel contacts was done by electron beam lithography. The layer of 8-Å-thick TiO 2 tunnel barrier was achieved by a twofold deposition of 4 Å Ti by electron beam evaporation and oxidation in oxygen atmosphere. Subsequently, a layer of 65 nm Co was deposited and capped with 4 nm Al. The Al oxidizes to form a native AlO x to protect the oxidation of Co contacts. Characterization of CVD graphene Atomic force microscope and Raman spectroscopy on the patterned CVD graphene were performed to optimize the fabrication process and ensure minimal residue accumulation during the processing. The quality of the TiO 2 /Co tunnel contacts was confirmed by three-terminal DC electrical measurements. The tunnel contacts showed resistances in the range 4–5 kΩ at room temperature, with a weak increase at 4.2 K. Gate voltage sweeps were done using a Keithley 2400 source meter in the range of ±40 V, to evaluate the square resistance and carrier mobility of graphene. Spin transport measurements Spin transport measurements in spin valve and Hanle configurations were performed using Keithley current source and nano-voltmeter in a variable temperature cryostat in liquid He/N 2 temperatures with a superconducting/electro magnets. We observed NL spin valve resistance (Δ R NL ) in the range 0.004–10 Ω, depending on the channel length, temperature and gate voltage. Evidence of spin signals for CVD graphene channel lengths longer than 16 μm, although found, were masked by the noise levels in our measurements. How to cite this article: Kamalakar, M. V. et al . Long-distance spin communication in chemical vapour-deposited graphene. Nat. Commun. 6:6766 doi: 10.1038/ncomms7766 (2015).